Structure and Scm3-mediated assembly of budding yeast centromeric nucleosomes Much controversy exists regarding the structural organization of the yeast centromeric nucleosome and the role of the nonhistone protein, Scm3, in its assembly and architecture. Here we show that the substitution of H3 with its centromeric variant Cse4 results in octameric nucleosomes that organize DNA in a left-handed superhelix. We demonstrate by single-molecule approaches, micrococcal nuclease digestion and small-angle X-ray scattering that Cse4-nucleosomes exhibit an open conformation with weakly bound terminal DNA segments. The Cse4-octamer does not preferentially form nucleosomes on its cognate centromeric DNA. We show that Scm3 functions as a Cse4-specific nucleosome assembly factor, and that the resulting octameric nucleosomes do not contain Scm3 as a stably bound component. Taken together, our data provide insights into the assembly and structural features of the budding yeast centromeric nucleosome. The centromere is a specific locus on each chromosome that directs the formation of the kinetochore, a multiprotein complex that interacts with spindle microtubules to promote proper chromosomal alignment and segregation during cell division [1] . The replacement of canonical (major-type) H3 with the centromere-specific histone variant CenH3 (known as CENP-A in humans and Cse4 in budding yeast) is essential for centromere function. CenH3 proteins from all organisms have a ∼ 90 amino-acid carboxy-terminal histone domain that exhibits ∼ 60% amino-acid sequence identity with canonical H3 ( Supplementary Fig. S1a ). Although canonical H3 is highly conserved between species, CenH3 is evolving rapidly [2] . The histone domain exhibits only 45–50% identity between various species, and its amino (N)-terminal tail is even more divergent in both length and amino-acid composition [3] . The protein composition, stoichiometry and structure of centromeric nucleosomes remain controversial. Mammalian centromeric nucleosomes are composed of two copies of each histone (CENP-A/H4/H2A/H2B) 2 (refs 4 , 5 , 6 ). Drosophila centromeric nucleosomes have been described as 'hemisomes' in vivo , containing only a single copy of each histone (CenH3/H4/H2A/H2B) [7] . In contrast, budding yeast centromeric nucleosomes are thought to form either octameric or hexameric complexes [8] , [9] , [10] . In the proposed hexameric structure, the two H2A/H2B dimers are replaced by the nonhistone protein Scm3 (ref. 11 ). In fission yeast, H2A/H2B dimers are depleted from the inner centromere regions containing CenH3 (ref. 12 ). Reports on the conformation of DNA in centromeric nucleosomes are also contradictory [5] , [13] . There is evidence from in vitro (Drosophila) and in vivo ( Saccharomyces cerevisiae ) experiments that the assembly of centromeric nucleosomes onto plasmid DNA induces positive supercoils [13] . This suggests that the DNA in centromeric nucleosomes is wrapped around the histone complex in a right-handed, as opposed to the canonical left-handed, superhelix. Because of obvious structural constraints [14] , the composition of these particles might be tetrameric or hexameric [13] , suggesting a third type of yeast centromeric 'nucleosome'. Structural and in vivo studies of human CENP-A show that the 22 amino-acid CENP-A-targeting domain is critical for its localization to the centromere [15] . The structure of the (CENP-A/H4) 2 tetramer—in the absence of DNA—revealed a high degree of similarity to major-type H3/H4 in a nucleosome. However, several unique features were noted [5] . As only two of the eight amino acids responsible for the unique structural features of the (CENP-A/H4) 2 tetramer are conserved in Cse4 ( Supplementary Fig. S1a ), the interpretations derived from the human (CENP-A/H4) 2 structure cannot easily be applied to the yeast (Cse4/H4) 2 tetramer. Budding yeast centromeres consist of a single 125 bp consensus sequence that is strictly required for centromere formation and that harbours a single Cse4-containing nucleosome [16] , [17] . The CEN regions of all 16 yeast centromeres all contain three consensus elements, termed CDE I, CDE II and CDE III [18] . The site of Cse4 occupancy is CDE II, a highly AT-rich (>90%) 78–86 bp DNA region [19] . CEN DNA-binding factor 3 (CBF3), binds to the CDE III consensus element, and the CDE III–CBF3 complex is required for centromere chromatin formation and function [20] . CDE I is the binding site for Cbf1 protein, which sharply bend the CEN DNA [18] . The interaction of CBF3 and Cbf1 with nucleosomal DNA may require special, as yet unidentified structural features of the Cse4-nucleosome. Moreover, the effect of this unusual DNA sequence on the structure, composition and stability of the centromeric yeast nucleosome has not been investigated. There is evidence that CenH3-specific factors deposit CenH3 at the appropriate location. In budding and fission yeast, this role is played by Scm3, a protein that is required for G2/M progression and incorporation of CenH3 to the centromere [8] , [11] , [12] , [21] , [22] . The functional mammalian homologue HJURP also has histone chaperone-like activity and facilitates deposition of the (CENP-A-H4) 2 tetramer onto DNA [23] , [24] , [25] . In budding yeast, Scm3 interacts directly with the Ndc10 subunit of the CBF3 complex [26] and depends on Ndc10 for its association with the centromere [21] . In vitro , Scm3 forms a stable complex with Cse4/H4 (refs 8 , 11 ) and displaces H2A/H2B dimers from refolded histone octamer [11] ; however, whether or not Scm3 is a permanent component of the centromeric 'nucleosome' remains controversial [8] , [11] . Here we present biochemical and biophysical studies that reveal structural features of budding yeast Cse4-nucleosomes and shed light on the function of Scm3 in nucleosome assembly. We find that the Cse4-nucleosome is composed of two copies each of Cse4, H4, H2A and H2B that organize DNA in a left-handed superhelix. The Cse4-nucleosome has an extended conformation due to weaker DNA–histone interactions in the peripheral region of the nucleosome. Cse4 does not intrinsically prefer its native CEN DNA. Moreover, we found that Scm3 is not an integral component of Cse4-nucleosmes; rather, it functions as a Cse4-specific nucleosome assembly factor. Cse4-nucleosomes exhibit an elongated structure To investigate the structural features of S. cerevisiae centromeric nucleosomes, we refolded recombinant yeast H2A, H2B and H4 with either recombinant H3 or its centromere-specific equivalent Cse4. Histone octamers with full-length or N-terminal tail deletions (Cse4 Δ102 , Cse4 Δ127 ) were also prepared. Cse4 Δ127 corresponds to the structured region of H3, whereas Cse4 Δ102 has an N-terminal tail that is similar in length to that of yeast H3 ( Supplementary Fig. S1a ). All histone octamers eluted at the expected volume from the gel-filtration column ( Supplementary Fig. S1b ) and contained equimolar amounts of the four histones ( Supplementary Fig. S1d ). Nucleosomes were reconstituted onto a 147 bp fragment derived from α-satellite DNA [27] by salt deposition, and analysed by native polyacrylamide gel electrophoresis (PAGE). Nucleosomes reconstituted from S. cerevisiae histones (Sc-Nuc) migrate similarly to nucleosomes made with Xenopus laevis histones (Xl-Nuc; Fig. 1a , lanes 3 and 6). In contrast, nucleosomes reconstituted with yeast H2A, H2B, H4 and Cse4 (Cse4-Nuc) migrate more slowly on native gels ( Fig. 1a , lane 2). This property is not a function of the extended N-terminal tail of Cse4, as partial or complete deletion of the Cse4 tail had little effect on gel migration ( Fig. 1a , compare lanes 4 and 5 with lane 2). Similar gel mobility properties were also observed for Cse4-nucleosomes reconstituted onto S. cerevisiae centromeric DNA (147-bp CEN3) and a 147 bp fragment of the '601' nucleosome positioning sequence (601 DNA) [28] ( Fig. 1a , compare lanes 7 and 8 with 10 and 11; See Supplementary Table S1 for all DNA sequences). 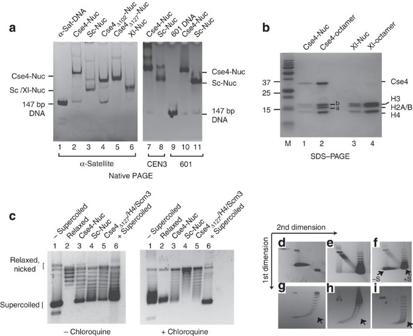Figure 1:In vitroassembled Cse4-containing nucleosomes exhibit retarded gel mobility and organize DNA in left-handed superhelix. (a) Cse4-nucleosomes were reconstituted onto 147-bp DNA segments by salt dilution and analysed by 5% native PAGE followed by ethidium bromide staining. Lane 1: 147-bp α-satellite DNA; lanes 2, 4 and 5: nucleosomes with full-length Cse4, Cse4Δ102and Cse4Δ127, respectively, assembled on α-sat DNA; lanes 3 and 6:S. cerevisiae(Sc) andXenopus laevis(Xl) nucleosomes on α-sat DNA, respectively. Lanes 7 and 8: Cse4- and Sc-nucleosomes reconstituted on yeast centromeric DNA (CEN3); lane 9: 147-bp 601 DNA; lanes 10 and 11: Cse4- and Xl-nucleosomes reconstituted on 147-bp 601 DNA. (b) Nucleosome bands were eluted from the gel shown ina, lanes 2 and 6, and analysed by SDS–PAGE and Coomassie Blue staining. Lanes 1 and 3: Cse4- and Xl-nucleosome bands; 2 and 4: Cse4- and Xl-octamers; M: protein molecular weight standards. Bands indicated as 'a': yeast H2A; 'b': yeast H2B. (c–i) Cse4-nucleosomes induce negative supercoiling: (c) Nucleosomes were assembled on a circular pBR322 plasmid using yNap1 in the presence of Topoisomerase I. Deproteinized DNA was analysed on 1.2% agarose gel in the absence (left panel) and presence of 2 μg ml−1chloroquine (right panel). Lane 1: negatively supercoiled plasmid; lane 2: relaxed plasmid; lanes 3 and 4: Cse4- and Sc-nucleosomes, respectively; lane 5: Cse4Δ127/H4/Scm3; lane 6: positively supercoiled pBR322 plasmid (purchased from Inspiralis). (d–i) Two-dimensional gel analysis of plasmid supercoiling. (d) and (e): negatively and positively supercoiled plasmid DNA, respectively, (f): samples ind,ecombined; plasmid supercoiling induced by Cse4-nucleosomes (g), Cse4Δ127/H4/Scm3/DNA complex (h) and Sc-nucleosomes (i). −S and +S refer to negatively and positively supercoiled plasmid DNA. The arrow ing–iindicates wherein the most supercoiled topoisomers run if they were positively supercoiled. We analysed the protein content of the main, most intense band for each nucleosome sample excised from the gel shown in Figure 1a . The reconstituted nucleosomes contained equimolar amounts of all four histones (Cse4, H4, H2A and H2B; Fig. 1b ). This was verified by size-exclusion chromatography coupled with multiangle light scattering (SEC–MALS). The molecular weight of all nucleosomes was fully consistent with a monodisperse complex of two copies of each histone and 147 bp of DNA ( Table 1 and Supplementary Fig. S2b ). Figure 1: In vitro assembled Cse4-containing nucleosomes exhibit retarded gel mobility and organize DNA in left-handed superhelix. ( a ) Cse4-nucleosomes were reconstituted onto 147-bp DNA segments by salt dilution and analysed by 5% native PAGE followed by ethidium bromide staining. Lane 1: 147-bp α-satellite DNA; lanes 2, 4 and 5: nucleosomes with full-length Cse4, Cse4 Δ102 and Cse4 Δ127 , respectively, assembled on α-sat DNA; lanes 3 and 6: S. cerevisiae (Sc) and Xenopus laevis (Xl) nucleosomes on α-sat DNA, respectively. Lanes 7 and 8: Cse4- and Sc-nucleosomes reconstituted on yeast centromeric DNA (CEN3); lane 9: 147-bp 601 DNA; lanes 10 and 11: Cse4- and Xl-nucleosomes reconstituted on 147-bp 601 DNA. ( b ) Nucleosome bands were eluted from the gel shown in a , lanes 2 and 6, and analysed by SDS–PAGE and Coomassie Blue staining. Lanes 1 and 3: Cse4- and Xl-nucleosome bands; 2 and 4: Cse4- and Xl-octamers; M: protein molecular weight standards. Bands indicated as 'a': yeast H2A; 'b': yeast H2B. ( c – i ) Cse4-nucleosomes induce negative supercoiling: ( c ) Nucleosomes were assembled on a circular pBR322 plasmid using yNap1 in the presence of Topoisomerase I. Deproteinized DNA was analysed on 1.2% agarose gel in the absence (left panel) and presence of 2 μg ml −1 chloroquine (right panel). Lane 1: negatively supercoiled plasmid; lane 2: relaxed plasmid; lanes 3 and 4: Cse4- and Sc-nucleosomes, respectively; lane 5: Cse4 Δ127 /H4/Scm3; lane 6: positively supercoiled pBR322 plasmid (purchased from Inspiralis). ( d – i ) Two-dimensional gel analysis of plasmid supercoiling. ( d ) and ( e ): negatively and positively supercoiled plasmid DNA, respectively, ( f ): samples in d , e combined; plasmid supercoiling induced by Cse4-nucleosomes ( g ), Cse4 Δ127 /H4/Scm3/DNA complex ( h ) and Sc-nucleosomes ( i ). −S and +S refer to negatively and positively supercoiled plasmid DNA. The arrow in g – i indicates wherein the most supercoiled topoisomers run if they were positively supercoiled. Full size image Table 1 Full size table We next wanted to examine whether the incorporation of Cse4 causes a reversal in the nucleosomal DNA superhelix handedness in Cse4-nucleosomes, as proposed previously [29] . Both Cse4- and Sc-nucleosomes were assembled onto relaxed plasmid DNA at low salt using the yeast histone chaperone Nap1 (yNap1). Assemblies were analysed by agarose gel electrophoresis in the absence and presence of chloroquine ( Fig. 1c ). The data show that both Sc- and Cse4-nucleosomes induce mainly negative supercoils. This was confirmed with a two-dimensional gel system first in the absence, then in the presence of chloroquine. This approach allows for the separation of mixtures of positively and negatively supercoiled DNA ( Fig. 1f–i ). Cse4- and Sc-nucleosomes exhibited identical behaviour ( Fig. 1g,i ), in that the vast majority of supercoiled plasmid fractions were negatively supercoiled. To further investigate the structural differences resulting from the incorporation of Cse4, we used small-angle X-ray scattering (SAXS). We compared Xl-, Sc- and Cse4-nucleosomes assembled on 147-bp 601 DNA. To minimize effects caused by the differences in tail length between yeast H3 and Cse4 ( Supplementary Fig. S1a ), we used the truncated version of Cse4 (Cse4 Δ102 ). As shown above, partial deletion of the Cse4 N-terminal tail does not significantly affect the slow gel migration signature of Cse4 Δ102 nucleosomes. All samples were shown to be monodisperse by native PAGE and SEC–MALS before data collection ( Supplementary Fig. S2a,b ). A comparison of the scaled intensity curves of the three nucleosomes indicates clear differences between Cse4 Δ102 -nucleosomes and canonical nucleosomes ( Fig. 2a ). The P(r) functions have the characteristic bell shape of globular complexes with well-defined maximum particle sizes for all three nucleosome preparations ( Fig. 2b ). The radius of gyration ( R g ) and maximum dimensions ( D max ) for Xl-nucleosomes were 41 and 120 Å, respectively ( Fig. 2b and Supplementary Table S2 ). The scattering curve calculated from the crystal structure (1kx5; ref. 30 ) superposes well with the experimental scattering curve of Xl-nucleosomes ( Fig. 2c ). The ab initio calculated envelope for Xl-nucleosome exhibits excellent shape and size correspondence with the crystal structure ( Supplementary Fig. S2c ). Sc-nucleosomes are characterized by a slightly increased R g ( ∼ 42.5 Å) and a D max of ∼ 135 Å, but the experimental scattering curve remains in close correspondence with the scattering curve calculated from the crystal structure ( Fig. 2d ); however, the envelope of Sc-nucleosome is somewhat extended ( Supplementary Fig. S2d ). The replacement of yeast H3 with Cse4 Δ102 resulted in an even more extended structure ( R g ∼ 46.5 Å; D max ∼ 165 Å; Fig. 2b and Supplementary Table S2 ), as well as in distinct differences in the intensity curves ( Fig. 2e ). The magnitude of the observed differences for nucleosomes with different conformations is consistent with those published earlier by us and others [31] , [32] . The calculated envelope for Cse4 Δ102 -nucleosomes can be fit with a nucleosome, but the envelope displays pronounced protrusions ( Supplementary Fig. S2e ). This is consistent with the slow gel mobility of Cse4-nucleosomes. Together, our data demonstrate that the incorporation of Cse4 results in nucleosomes that organize DNA in a canonical negative supercoil around a histone octamer, and that these nucleosomes are somewhat extended. 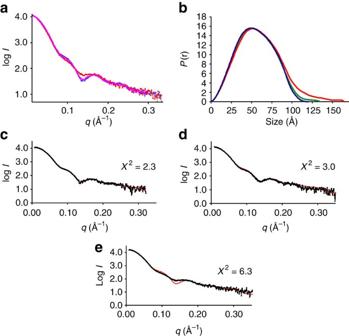Figure 2: Cse4-nucleosomes exhibit an extended morphology. (a) Normalized SAXS curves of nucleosomes. Cse4Δ102-nucleosomes (red) produce a clearly different scattering curve compared with Sc-nucleosomes (magenta) or Xl-nucleosomes (blue). (b) Distance distribution functions (P(r)) of the three nucleosomes shown ina. Xl-nucleosome is shown in blue, Sc-nucleosome in green and Cse4Δ102-nucleosomes in red. Differences in the maximum dimensions of the three nucleosomes (see alsoSupplementary Table S2) are obvious.Ab initioenvelopes, calculated from the intensity data, are shown inSupplementary Figure S2. (c–e) Comparison of experimental scattering profiles (black) with a scattering profile calculated using FoXS51from the Xl-nucleosome crystal structure (1kx5; red). Experimental profiles from Xl-, Sc- and Cse4Δ102-nucleosomes are inc–e, respectively. Theχ2values of the fit between the two curves are shown. Figure 2: Cse4-nucleosomes exhibit an extended morphology. ( a ) Normalized SAXS curves of nucleosomes. Cse4 Δ102 -nucleosomes (red) produce a clearly different scattering curve compared with Sc-nucleosomes (magenta) or Xl-nucleosomes (blue). ( b ) Distance distribution functions ( P (r)) of the three nucleosomes shown in a . Xl-nucleosome is shown in blue, Sc-nucleosome in green and Cse4 Δ102 -nucleosomes in red. Differences in the maximum dimensions of the three nucleosomes (see also Supplementary Table S2 ) are obvious. Ab initio envelopes, calculated from the intensity data, are shown in Supplementary Figure S2 . ( c – e ) Comparison of experimental scattering profiles (black) with a scattering profile calculated using FoXS [51] from the Xl-nucleosome crystal structure (1kx5; red). Experimental profiles from Xl-, Sc- and Cse4 Δ102 -nucleosomes are in c – e , respectively. The χ 2 values of the fit between the two curves are shown. Full size image The Cse4-nucleosome organizes only 115 bp of DNA The observed characteristics of the Cse4-nucleosome could be because of less tightly bound DNA at the entry/exit regions. To test this, micrococcal nuclease (MNase) digestion of Cse4- and Sc-nucleosomes was conducted. Nucleosomes were reconstituted on either a linearized plasmid DNA using Nap1 or onto a 147-bp 601 DNA fragment by salt dilution. Cse4-nucleosomes offer less resistance towards MNase digestion than do Sc-nucleosomes, and protect only ∼ 110–120 bp of DNA ( Supplementary Fig. S3 ). This finding correlates with a recent report, wherein salt-reconstituted Cse4 nucleosomes were shown to protect ∼ 125 bp [33] . We used a single-molecule DNA-unzipping approach to provide a direct comparison of histone-DNA interactions in a Cse4-nucleosome compared with an Sc-nucleosome. A DNA molecule containing either a single Cse4- or Sc-nucleosome assembled onto 601 DNA was attached to the surface of a microscope coverslip via one of its strands and to a microsphere held in an optical trap via the other strand ( Supplementary Fig. S4 ). The magnitude of resistance towards unzipping strongly correlates with the strength of histone-DNA interactions, and thus a histone-DNA interaction map can be generated along the DNA [34] . We first examined Sc-nucleosomes by unzipping DNA from either the forward or reverse direction along the DNA sequence ( Fig. 3 , left panel). Two distinct regions of interactions were detected; contacts between the H2A/H2B dimers and the DNA (super-helical location (SHL) ∼ ±3.5 to ±6.5); and contacts between the (H3/H4) 2 tetramer and the DNA (SHL ∼ −2.5 to +2.5). Within each region, interactions were discretely spaced with ∼ 5 bp periodicity ( Supplementary Figs S5 and 6 ). Signatures from recombinant yeast nucleosomes are indistinguishable from those obtained with nucleosomes from native HeLa histones [34] . Unzipping through a DNA molecule assembled with a tetramer exhibited only a single region of interaction that substantially overlapped with the SHL −2.5 to 2.5 region where (H3/H4) 2 tetramer contacts DNA in canonical nucleosomes ( Supplementary Fig. S5 ). 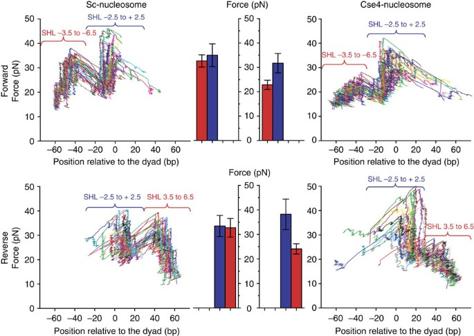Figure 3: Single-molecule analysis shows that Cse4-nucleosomes have weakened histone–DNA interactions in the peripheral regions. Nucleosome disruption signatures under a constant loading rate (8 pN s−1). Representative traces are shown for canonical Sc-nucleosomes (left panel) and Cse4-nucleosomes (right panel), where each colour represents data obtained from a single-nucleosomal DNA molecule. Interaction regions are defined according to the crystal structure27as super-helical location (SHL) −2.5 to +2.5 (H3/H4 tetramer interaction region) and SHL ±3.5 to ±6.5 (H2A/H2B dimer interaction region). Within the SHL −2.5 to +2.5 region the maximum disruption forces observed are similar between Sc- and Cse4-nucleosomes. Cse4-nucleosomes have significantly weaker interactions throughout the peripheral regions (SHL ±3.5 to ±6.5). A quantitative comparison of the peak forces measured within each interaction region is shown (centre panel). SHL ±3.5 to ±6.5 is shown in red bar and SHL −2.5 to +2.5 shown in blue. Error bars represent s.d. SeeSupplementary Figures S4–6for additional data. Figure 3: Single-molecule analysis shows that Cse4-nucleosomes have weakened histone–DNA interactions in the peripheral regions. Nucleosome disruption signatures under a constant loading rate (8 pN s −1 ). Representative traces are shown for canonical Sc-nucleosomes (left panel) and Cse4-nucleosomes (right panel), where each colour represents data obtained from a single-nucleosomal DNA molecule. Interaction regions are defined according to the crystal structure [27] as super-helical location (SHL) −2.5 to +2.5 (H3/H4 tetramer interaction region) and SHL ±3.5 to ±6.5 (H2A/H2B dimer interaction region). Within the SHL −2.5 to +2.5 region the maximum disruption forces observed are similar between Sc- and Cse4-nucleosomes. Cse4-nucleosomes have significantly weaker interactions throughout the peripheral regions (SHL ±3.5 to ±6.5). A quantitative comparison of the peak forces measured within each interaction region is shown (centre panel). SHL ±3.5 to ±6.5 is shown in red bar and SHL −2.5 to +2.5 shown in blue. Error bars represent s.d. See Supplementary Figures S4–6 for additional data. Full size image The unzipping signature of Cse4-nucleosomes resembles that of Sc-nucleosomes ( Fig. 3 , right panel and Supplementary Fig. S6 ). However, the peak forces in SHL 3.5–6.5 regions in both sides of the nucleosomes were significantly lower than those of Sc-nucleosomes, suggesting that the DNA is more weakly bound to this region of the Cse4 histone octamer. Unexpectedly, the histone–DNA interactions in SHL ∼ −2.5 to 2.5 region (flanking the dyad by ∼ 30 bp), which involves the majority of direct contributions from H3 or Cse4, is at least as tight as in Sc-nucleosomes ( Fig. 3 ). The force required for the unzipping fork to overcome the second region from the reverse direction is slightly higher for Cse4-nucleosomes, indicating a small asymmetric Cse4-induced increase in interaction strength at the tetramer. Taken together, this indicates that the overall structure of a centromeric nucleosome resembles that of a canonical nucleosome except for the more loosely bound outer ∼ 2×2=40 bp of DNA. Cse4-octamers do not preferentially assemble on CEN3 DNA S. cerevisiae centromeric DNA is highly AT-rich, making it a poor substrate for nucleosome formation [35] . Nevertheless, Cse4- and Sc-nucleosomes can be reconstituted on CEN3 DNA ( Fig. 1a , lanes 7 and 8). We wanted to examine whether Cse4-octamers preferentially assemble on CEN3 DNA. Using salt deposition, we reconstituted a limiting amount of histone octamers on a cy3-labelled 207-bp 601 or atto647-labelled 207-bp CEN3 DNA fragment in the presence of an excess of unlabelled 147-bp 5S DNA (see experimental scheme in Fig. 4a ). The fraction of DNA incorporated into nucleosomes (using data from Fig. 4b–d with histone–DNA ratio of 0.32:1 for Cse4-octamer, and 0.28:1 for Sc-octamer) was quantified ( Fig. 4e ). Both Cse4- and Sc-octamers preferentially assemble on 601 DNA compared with 5S DNA, confirming the strong positioning propensities of this sequence [28] . Both octamers assembled much less efficiently on CEN3 DNA and 5S DNA, demonstrating that the Cse4-octamer does not have an intrinsic preference for its native CEN DNA. 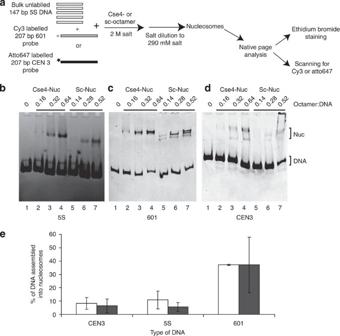Figure 4: Cse4-nucleosomes do not preferentially assemble on CEN3 DNA. (a) Experimental scheme of Cse4- and Sc-nucleosomes reconstitution on 5S, 601 and CEN3 DNA. Nucleosomes were reconstituted under limiting octamer concentration by salt dilution on either a 207-bp atto647-labelled CEN3 or cy3-labelled 601 DNA probe in the presence of an excess of 147-bp 5S DNA and analysed by 5% native PAGE. (b) The reconstitution on total DNA (≈5S DNA) was visualized by ethidium bromide staining. Nucleosomes assembled on 601 DNA and CEN3 DNA were detected by scanning for cy3 601 (c) and atto647 (d), respectively. The ratio of octamer to DNA and the types of histone octamer (Cse4, Sc) used are indicated above the lanes. (e) Quantification of nucleosome assembly. The fraction of DNA incorporated into nucleosomes inb–dwas calculated by dividing the signal of the shifted band(s) by the sum of free DNA and shifted band signal, and multiplying by 100. We excluded the material in the wells, but added all nucleosome bands. The graph of nucleosomes reconstituted using octamer–DNA ratio of 0.32:1 (Cse4-Nuc, shown in white) and 0.28:1 (Sc-nuc, shown in black) is shown. The mean and standard deviation values from 4 to 5 different experiments were used to plot the graph. Figure 4: Cse4-nucleosomes do not preferentially assemble on CEN3 DNA. ( a ) Experimental scheme of Cse4- and Sc-nucleosomes reconstitution on 5S, 601 and CEN3 DNA. Nucleosomes were reconstituted under limiting octamer concentration by salt dilution on either a 207-bp atto647-labelled CEN3 or cy3-labelled 601 DNA probe in the presence of an excess of 147-bp 5S DNA and analysed by 5% native PAGE. ( b ) The reconstitution on total DNA (≈5S DNA) was visualized by ethidium bromide staining. Nucleosomes assembled on 601 DNA and CEN3 DNA were detected by scanning for cy3 601 ( c ) and atto647 ( d ), respectively. The ratio of octamer to DNA and the types of histone octamer (Cse4, Sc) used are indicated above the lanes. ( e ) Quantification of nucleosome assembly. The fraction of DNA incorporated into nucleosomes in b – d was calculated by dividing the signal of the shifted band(s) by the sum of free DNA and shifted band signal, and multiplying by 100. We excluded the material in the wells, but added all nucleosome bands. The graph of nucleosomes reconstituted using octamer–DNA ratio of 0.32:1 (Cse4-Nuc, shown in white) and 0.28:1 (Sc-nuc, shown in black) is shown. The mean and standard deviation values from 4 to 5 different experiments were used to plot the graph. Full size image To address the relative stability of Cse4- and Sc- nucleosomes reconstituted on various DNA fragments, we assayed their integrity after storage on ice for at least 24 h ( Supplementary Fig. S7 ). Cse4- and Sc-nucleosomes are equally stable when reconstituted on 601 DNA, and display no signs of dissociation after 1 week of storage on ice ( Supplementary Fig. S7a ). Similarly, Cse4-nucleosome reconstituted onto a generic 147-bp DNA fragment derived from pBR322 remains intact on storage ( Supplementary Fig. S7d ). In contrast, a Cse4-nucleosome reconstituted on its cognate CEN-DNA dissociates almost completely after 24 h of storage, whereas a Sc-nucleosome on the same DNA or a Cse4-nucleosome on 5S DNA remains largely intact ( Supplementary Fig. S7b,c ). Together, this data suggests that Cse4 and CEN DNA might have co-evolved to be particularly unstable in the absence of other centromere-specific factors. Scm3 is not a component of the Cse4-nucleosome It has been proposed that the putative centromeric histone chaperone Scm3 replaces histones H2A/H2B dimers in a Cse4-containing nucleosome-like particle. Scm3 can be refolded with Cse4 and H4 into a well-defined and monodisperse complex (ref. 11 and Supplementary Fig. S1c,d ). We tested whether this Cse4 Δ127 /H4/Scm3 complex can be reconstituted into Scm3-containing nucleosome-like particles. The refolded Cse4 Δ127 /H4/Scm3 complex was reconstituted on 207-bp 601 DNA using salt dilution. The resulting species exhibited variable electrophoretic mobility ( Fig. 5a ). The major (and in case of lane 5, minor) bands were eluted from the gel and analysed by SDS–PAGE ( Fig. 5b ). Only (Cse4 Δ127 /H4) 2 , but not Scm3, is bound to DNA in any of these complexes ( Fig. 5b , lanes 6 and 7). When the same reaction was repeated in the presence of H2A/H2B dimer, an octameric nucleosome complex consisting of Cse4, H4, H2A and H2B was formed (data not shown). 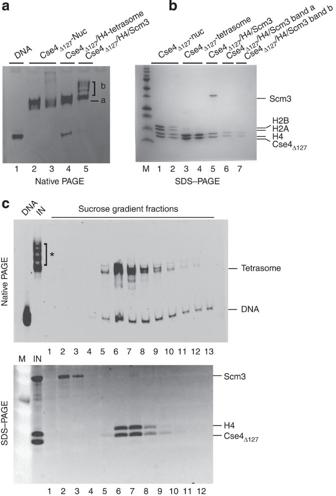Figure 5: Scm3 is not stably incorporated into nucleosome-like particles. (a) Two different concentrations of Cse4Δ127-octamer (lanes 2 and 3), (Cse4Δ127/H4)2tetramer (lane 4) and Cse4Δ127/H4/Scm3 (lane 5) were reconstituted on 601 DNA (207 bp) by salt dilution and analysed by gel-shift on native 5% PAGE. In lane 5, 'a' and 'b' refer to the lower discrete band and upper multiple bands, respectively. (b) Individual bands from gel shown inawere excised and analysed by 16% SDS–PAGE. Lanes 1: control Cse4Δ127-nucleosome; 2: Cse4Δ127-nucleosome band (from lane 3 ina); 3: control (Cse4Δ127/H4)2tetrasome; 4: (Cse4Δ127/H4)2tetrasome band (lane 4 ina); 5: control Cse4Δ127/H4/Scm3 complex; 6 and 7 correspond to the bands labelled as 'a' and 'b', respectively from lane 5 ina. (c) Sucrose density gradient fractionation of Cse4Δ127/H4/Scm3 reconstituted on 601, 207 bp DNA. Samples were fractionated in a 5–25% sucrose density gradient. Upper panel: the fractions were analysed on 5% native PAGE and stained with ethidium bromide. Lanes: DNA: 207-bp 601; IN, input sample; 1–13: fractions from low- to high-density sucrose. Lower panel: samples 1–12 shown in the upper panel were analysed by SDS–PAGE stained with SYPRO Ruby (Invitrogen). Figure 5: Scm3 is not stably incorporated into nucleosome-like particles. ( a ) Two different concentrations of Cse4 Δ127 -octamer (lanes 2 and 3), (Cse4 Δ127 /H4) 2 tetramer (lane 4) and Cse4 Δ127 /H4/Scm3 (lane 5) were reconstituted on 601 DNA (207 bp) by salt dilution and analysed by gel-shift on native 5% PAGE. In lane 5, 'a' and 'b' refer to the lower discrete band and upper multiple bands, respectively. ( b ) Individual bands from gel shown in a were excised and analysed by 16% SDS–PAGE. Lanes 1: control Cse4 Δ127 -nucleosome; 2: Cse4 Δ127 -nucleosome band (from lane 3 in a ); 3: control (Cse4 Δ127 /H4) 2 tetrasome; 4: (Cse4 Δ127 /H4) 2 tetrasome band (lane 4 in a ); 5: control Cse4 Δ127 /H4/Scm3 complex; 6 and 7 correspond to the bands labelled as 'a' and 'b', respectively from lane 5 in a . ( c ) Sucrose density gradient fractionation of Cse4 Δ127 /H4/Scm3 reconstituted on 601, 207 bp DNA. Samples were fractionated in a 5–25% sucrose density gradient. Upper panel: the fractions were analysed on 5% native PAGE and stained with ethidium bromide. Lanes: DNA: 207-bp 601; IN, input sample; 1–13: fractions from low- to high-density sucrose. Lower panel: samples 1–12 shown in the upper panel were analysed by SDS–PAGE stained with SYPRO Ruby (Invitrogen). Full size image To exclude the possibility that Scm3 dissociated from the complex during gel electrophoresis, we examined the products of salt-mediated Cse4 Δ127 /H4/Scm3/DNA reconstitution by sucrose gradient sedimentation analysis. The slow migrating bands (indicated by '*') were not stable and dissociated during sedimentation ( Fig. 5c upper panel); these bands are likely additional Cse4 Δ127 /H4 in loose association with the Cse4 Δ127 /H4/DNA complex (tetrasome). (Cse4 Δ127 /H4) 2 tetrasome and Scm3 elute separately in the sucrose gradient ( Fig. 5c lower panel), confirming that Scm3 is not stably associated with the Cse4 Δ127 /H4/DNA complex. Control Cse4 Δ127 -nucleosomes reconstituted on the same DNA contained all four histones (Cse4 Δ127 , H4, H2A and H2B; Supplementary Fig. S8 ), demonstrating that the Cse4 Δ127 -nucleosomes were stable during sucrose gradient sedimentation. We also investigated the superhelical organization of particles reconstituted from refolded Cse4 Δ127 /H4/Scm3 using a plasmid supercoiling assay. This complex introduced predominantly negative supercoils into plasmid DNA ( Fig. 1c , lane 5 in left and right panels, and Fig. 1h ). This shows that the canonical handedness of the DNA supercoil is maintained even in the absence of H2A/H2B dimer and in presence of Scm3. Scm3 functions as a Cse4-specific nucleosome assembly factor Scm3 is required for CenH3 deposition on the centromere in both S. cerevisiae and Schizosaccharomyces pombe [11] , [12] , [21] , [22] . We investigated whether Scm3 mediates Cse4-nucleosome assembly in vitro. We also wanted to exclude the possibility that under these physiological (as opposed to high-ionic strength) conditions Scm3 remains an integral part of the yeast centromeric nucleosome [10] ), perhaps altering the handedness of the resulting nucleosomes, as observed in vivo [13] . We expressed a truncated version of Scm3, encompassing the conserved Cse4-binding region of Scm3 (amino acids 63–189; Scm3 63–189 ) [11] , [36] and full-length Scm3 in Escherichia coli ( Supplementary Fig. S1e ). In our standard chaperone-mediated chromatin assembly assay, we used Scm3 or Scm3 63–189 (in place of yNAP1) on a plasmid containing four copies of 190-bp CEN3 and four copies of CEN, followed by an analysis of supercoiling ( Fig. 6a ). 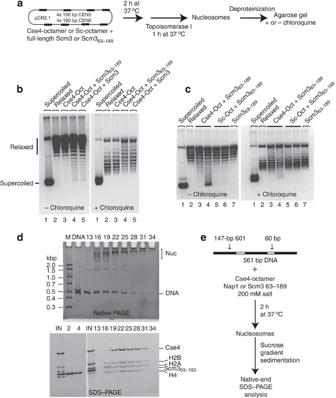Figure 6: Scm3 is a Cse4-specific chaperone that assembles nucleosomes with a negative supercoil. (a) As illustrated in the schematic, Cse4- or Sc-nucleosomes were assembled on relaxed circular plasmid DNA using full-length Scm3 or truncated Scm363–189as a histone chaperone; nucleosome assembly was analysed by plasmid supercoiling assay. (b,c) Deproteinized DNA samples were analysed on 1% agarose gel in the absence and presence of chloroquine (as indicated), and visualized by SYBR Gold staining. (b) Full-length Scm3 and Scm363–189assemble nucleosomes equally well. Lanes 1 and 2: negatively supercoiled or relaxed pCR2.1-(CEN3+CEN6)4; lane 3: Cse4-octamer (Oct) without histone chaperone; lanes 4 and 5: Cse4-octamer with 25 pmol Scm363–189and full-length Scm3, respectively. (c) Scm3 is specific for the Cse4-octamer: Cse4- or Sc-nucleosomes were assembled and analysed as described ina. Lanes 1 and 2: negatively supercoiled and relaxed plasmid, respectively; lanes 3 and 4: Cse4-nucleosome assembled in the presence of 25 and 50 pmol of Scm363–189, respectively; lanes 5 and 6: Sc-nucleosomes assembled in the presence of 25 and 50 pmol Scm363–189, respectively; lane 7: 50 pmol Scm363–189, no histone octamer. (d) Cse4-nucleosomes assembled by Scm3 contain all four histones but not Scm3: As diagramed ine, Cse4-nucleosomes were reconstituted on a 561-bp DNA containing three 147-bp 601 nucleosome positioning sequences using Scm363–189as the chromatin assembly factor. The assembled chromatin was purified by sucrose gradient sedimentation. Incremental fractions 13–34 (top to bottom of the sucrose gradient) were analysed by 4% native PAGE and visualized by ethidium bromide (upper panel). Input samples and fractions 2, 4, and incremental fractions13–34 were analysed by SDS–PAGE stained with SYPRO Ruby (Invitrogen; lower panel). Control experiments with Nap1 instead of Scm363–189as the assembly factor and assembly by full-length Scm3, and assembly on 207-bp CEN3 and 5S DNA by Scm363–189are shown inSupplementary Figure S9. (e) Experimental scheme of nucleosome reconstitution for data shown ind. Figure 6: Scm3 is a Cse4-specific chaperone that assembles nucleosomes with a negative supercoil. ( a ) As illustrated in the schematic, Cse4- or Sc-nucleosomes were assembled on relaxed circular plasmid DNA using full-length Scm3 or truncated Scm3 63–189 as a histone chaperone; nucleosome assembly was analysed by plasmid supercoiling assay. ( b , c ) Deproteinized DNA samples were analysed on 1% agarose gel in the absence and presence of chloroquine (as indicated), and visualized by SYBR Gold staining. ( b ) Full-length Scm3 and Scm3 63–189 assemble nucleosomes equally well. Lanes 1 and 2: negatively supercoiled or relaxed pCR2.1-(CEN3+CEN6) 4 ; lane 3: Cse4-octamer (Oct) without histone chaperone; lanes 4 and 5: Cse4-octamer with 25 pmol Scm3 63–189 and full-length Scm3, respectively. ( c ) Scm3 is specific for the Cse4-octamer: Cse4- or Sc-nucleosomes were assembled and analysed as described in a . Lanes 1 and 2: negatively supercoiled and relaxed plasmid, respectively; lanes 3 and 4: Cse4-nucleosome assembled in the presence of 25 and 50 pmol of Scm3 63–189 , respectively; lanes 5 and 6: Sc-nucleosomes assembled in the presence of 25 and 50 pmol Scm3 63–189 , respectively; lane 7: 50 pmol Scm3 63–189 , no histone octamer. ( d ) Cse4-nucleosomes assembled by Scm3 contain all four histones but not Scm3: As diagramed in e , Cse4-nucleosomes were reconstituted on a 561-bp DNA containing three 147-bp 601 nucleosome positioning sequences using Scm3 63–189 as the chromatin assembly factor. The assembled chromatin was purified by sucrose gradient sedimentation. Incremental fractions 13–34 (top to bottom of the sucrose gradient) were analysed by 4% native PAGE and visualized by ethidium bromide (upper panel). Input samples and fractions 2, 4, and incremental fractions13–34 were analysed by SDS–PAGE stained with SYPRO Ruby (Invitrogen; lower panel). Control experiments with Nap1 instead of Scm3 63–189 as the assembly factor and assembly by full-length Scm3, and assembly on 207-bp CEN3 and 5S DNA by Scm3 63–189 are shown in Supplementary Figure S9 . ( e ) Experimental scheme of nucleosome reconstitution for data shown in d . Full size image Scm3 clearly assembles Cse4-nucleosomes, and the conserved region (Scm3 63–189 ) is sufficient for this activity ( Fig. 6b left panel, compare lanes 4 and 5). Scm3 63–189 is specific for Cse4, as it showed only poor assembly of Sc-nucleosomes ( Fig. 6c left panel)). As observed for Cse4-nucleosomes assembled by yNap1 ( Fig. 1c ), Cse4-nucleosomes reconstituted with Scm3 and Scm3 63–189 induced negative DNA supercoils into plasmids containing CEN sequences ( Fig. 6b,c , right panels). Together, this data demonstrate that Scm3 has Cse4-specific histone chaperone activity that assembles nucleosomes with a left-handed DNA supercoil. As shown above ( Fig. 1a,b and Table 1 ), Cse4-nucleosomes reconstituted by a salt dilution approach in the absence of Scm3 are octameric in composition. We wanted to compare the composition of Cse4-nucleosomes reconstituted with yNap1 and Scm3 under physiological ionic strength onto different DNA sequences (601, 5S, CEN3). Cse4-octamers were assembled onto linear 561-bp DNA (containing three 147-bp 601 segments connected by 60-bp linker DNA) in the presence of yNap1, Scm3 63–189 or Scm3. The assembled nucleosomes (likely a mixture between mono-, di- and trinucleosomes) were fractionated by sucrose gradient sedimentation and the fractions were analysed by native PAGE and SDS–PAGE ( Fig. 6d,e and Supplementary Fig. S9 ). SDS–PAGE analysis of individual fractions demonstrates that Cse4-nucleosomes assembled on 601 DNA by yNap1 ( Supplementary Fig. S9a ), Scm3 ( Supplementary Fig. S9b ) or Scm3 63–189 ( Fig. 6d ) are composed of Cse4, H2A, H2B and H4. Neither yNap1, nor Scm3 or Scm3 63–189 co-fractionate with the nucleosome; both chaperones elute at significantly lower sucrose density and clearly separate from the nucleosomes. The yNap1 fractions that partially overlap with the nucleosome ( Supplementary Fig. S9a , right panel, lane 13 and 16) are likely caused by the previously described oligomerization of yNap1 dimers at physiological ionic strength [37] . Cse4-nucleosomes were also assembled on 207-bp CEN3 and 207-bp 5S DNA fragments using Scm3 63–189 as the assembly factor and were shown to be octameric ( Supplementary Fig. S9c,d ). Together, our results suggest that under the conditions used, Scm3 is not integrated into Cse4-nucleosomes on any of the DNA sequences tested, including CEN DNA. Thus, we conclude that Scm3 is not a stable component of Cse4-nucleosomes but functions as Cse4-nucleosome-specific assembly factor. Here we have shown that Cse4-nucleosomes resemble canonical nucleosomes in their octameric histone composition and DNA organization into a left-handed DNA supercoil, as shown recently by analytical ultra centrifuge and atomic force microscope [33] . The intrinsic properties of Cse4-containing histone complexes are sufficient to determine these features, as salt- and chaperone-mediated assembly pathways on different DNA sequences (including CEN DNA) have the same outcome. The unique sequence features of CEN DNA do not confer preference for Cse4. Under no condition do we observe a nucleosome-like particle consisting of Cse4, H4 and Scm3; rather our results suggest a role for Scm3 as a Cse4-specific assembly factor. Despite the overall similarities, we observe significant structural deviations in Cse4-nucleosomes. They exhibit an open conformation that is at least partly due to weaker interactions in the DNA regions organized by the H2A/H2B dimers, and by the N-terminal α-helix and the base of the N-terminal tail of Cse4. DNA sequences with poly (dA:T) tracts (as in CEN DNA) are predicted to disfavour the formation of stable nucleosomes [35] . We demonstrate that the Cse4-octamer does not exhibit a preference for CEN DNA, confirming interpretations from single-molecule experiments [38] . From their electrophoretic mobility, we surmise that Cse4-nucleosomes on CEN DNA also exist in the more open state observed for Cse4-nucleosomes on 601 and α-sat DNA. Cse4-nucleosomes on CEN3 DNA are particularly unstable on storage, and this may partly explain previous reports that Cse4-nucleosomes cannot be assembled on CEN DNA in vitro [8] , as well as the observed depletion of H2A/H2B, perhaps during preparation, from centromeric nucleosomes [11] . Thus, if there is a role for CEN DNA in modulating nucleosome structure at the yeast centromere, it is unlikely that it directly attracts (Cse4/H4) 2 , or that it forms particularly stable nucleosomes. Rather, the low propensity to form nucleosomes on CEN DNA suggests that centromeric sequences might have evolved to exclude any nucleosome formation to prevent incorporation of the abundant major-type H3. This allows for the targeted assembly of Cse4-nucleosomes only in the presence of centromeric proteins that are specific for Cse4 and CEN DNA. For example, the CBF3 complex interacts with Cbf1 and such interactions may be important to stabilize the observed 'open' centromeric nucleosomes. Thus, it seems that Cse4 has evolved to form a particularly unstable nucleosome on CEN DNA that is viable only in the presence of other key factors, ensuring proper centromere architecture. On the other hand, the more open architecture of Cse4-nucleosomes might generate an environment that is required for concurrent binding of centromere-associated proteins. Both CDE III and CDE I (the binding sites of CBF3 and Cbf1, respectively) are part of the 125-bp nucleosomal centromeric DNA. Assuming that Cse4-nucleosomes are also octameric in vivo [8] , partial dissociation of DNA ends would be required to allow binding of both CBF3 and Cbf1, as well as of other centromeric proteins (Scm3 and Mif2). This may serve as the foundation of kinetochore assembly. Our results favour a role for S. cerevisiae Scm3 as a Cse4/H4-specific assembly factor but not as a component of the Cse4-nucleosome. As the effects of scm3 deletion can be rescued by overexpression of Cse4 (ref. 8 ), it is possible that Nap1 (which assembles Cse4 and H3-containing histone octamers equally well) or another chaperone replaces Scm3 in its Cse4-nucleosome assembly function. The structural basis for Scm3 specificity for (Cse4/H4) 2 tetramer or in Cse4-nucleosome assembly needs further investigation. It has been suggested that Scm3 might displace H2A/H2B dimers from a Cse4-nucleosome to form (Scm3/Cse4/H4)-containing 'hexasomes' [11] , [38] . We have shown that Scm3 does not remain associated with DNA when refolded Scm3/Cse4/H4 complex is reconstituted onto DNA using salt dialysis, and that addition of H2A/H2B dimers to this reaction results in the formation of octameric nucleosomes. Octameric nucleosomes were also obtained when Scm3 was used as histone chaperone to assemble Cse4-nucleosomes under physiological salt conditions. Together, our data favour a model in which Scm3 interacts with CBF3 and other centromeric proteins to facilitate the deposition of Cse4/H4 on CEN DNA, resulting in the formation of an octameric Cse4-nucleosome. Once assembled, the intrinsic features of the Cse4-nucleosome on CEN DNA likely ensure that Cse4-nucleosomes (and not H3-nucleosomes) are only stable in the presence of other centromere-specific factors, ensuring proper centromere function. DNA preparation The various DNA sequences used for nucleosome reconstitution are listed in Supplementary Table S1 . The DNA fragments were prepared by cutting the appropriate plasmids with the appropriate restriction enzymes or by PCR. α-Satellite DNA (147 bp) was prepared as previously reported [39] . Protein purification and refolding A pKS387-Cse4 pET expression plasmid with a mutation in the Nde I site was a kind gift from the Harrison Laboratory. N-terminally truncated Cse4 constructs (Cse4 103–229 and Cse4 128–229) were PCR amplified from pKS387-Cse4, and inserted into Nde I/ Bam HI sites of pKS387-Cse4 plasmid replacing the full-length Cse4-coding sequence. Cse4 103–229 (Cse4 Δ102 ) lacks the N-terminal 102 amino acids; the remaining N-terminal tail is 9 amino acids shorter than that of canonical H3, whereas Cse4 128–229 (Cse4 Δ127 ) is the equivalent of tailless canonical H3. The Scm3-coding sequence was PCR amplified from yeast genomic DNA, and inserted into Bsp HI/ Eco RI sites of pHAT2 plasmid vector DNA resulting in the addition of His 6 to the N-terminus. Similarly, the coding region for Scm3 63–189 was cloned into a pHAT4 plasmid vector and the protein was expressed with an N-terminal His 6 -tag with a TEV cleavage site for removal of the tag. Recombinant Cse4 and other yeast histone proteins were expressed in E. coli and purified as described previously [40] . Full-length Scm3 was purified from inclusion bodies using published procedures [40] except that Q-sepharose (HiTrap Q FF, GE Healthcare) was used in the last step. Refolding of major-type and Cse4-containing histone octamers and tetramers, and of Cse4/H4/Scm3 complexes was done as described [40] . The full-length Scm3 was refolded in absence of Cse4 and H4 into a soluble state. Briefly, purified Scm3 was dissolved in buffer composed of 7 M guanidine-HCl, 20 mM Tris-HCl pH 8, 1 mM EDTA, 5 mM dithiothreitol (DTT), 20%glycerol and 0.01% NP40. The sample was then dialysed against buffer consisting of 20 mM Tris-HCl pH 8, 0.24 mM tris (2-carboxyethyl) phosphine, 300 mM NaCl, 0.2 mM PMSF, 0.3 mM benzamidine, 20% glycerol and 0.01% NP40. Truncated His 6 -tagged Scm3 63–189 was purified by Ni-NTA under native conditions. The His 6 -tag was removed with TEV protease, and the protein was further purified by gel-filtration using Superdex 75 in buffer containing 20 mM Tris-HCl pH 8, 300 mM NaCl, 1 mM pepstatin, 0.2 mM PMSF, 1 mM benzamidin and 0.01% NP40. The salt concentration was adjusted to 50 mM and was further purified over a HiTrap Q FF column (GE Healthcare). Nucleosome reconstitution by salt dilution Cse4-, Xenopus laevis (Xl-) and S. cerevisiae (Sc-) nucleosomes were reconstituted on 147- and 207-bp DNA (5S, 601, CEN3, pBR322 DNA; sequences given in the Supplementary Table S1 ) using standard salt dilution or dialysis [40] , and analysed by 5% native PAGE and ethidium bromide staining. The histone composition of Cse4-nucleosomes was determined by electro-eluting the nucleosome bands from a native PAGE, and examining their composition by SDS–PAGE. The stability of Cse4-nucleosome was determining by analysing nucleosome sample stored at 4 °C for 24 h or longer. Competitive nucleosome reconstitution Cse4-octamer (1.2–4.8 μg) or Sc-octamer (1.05–4.2 μg) was reconstituted by salt dilution onto 7.5 μg 146-bp 5S DNA in the presence of limiting amounts ( ∼ 200 ng) of Cy3-labelled 207-bp 601 DNA or Atto647-labelled CEN3 DNA. The samples were separated on a 5% native PAGE and visualized by ethidium bromide staining or scanned for fluorescence at the appropriate wavelength. The propensity of nucleosome formation on the different DNA sequences was determined by quantifying the percentage of 5S DNA or labelled DNA probe incorporated into nucleosomes. Histone chaperone-mediated nucleosome reconstitution Nucleosomes were reconstituted on relaxed circular plasmid or linear DNA using a histone chaperone [41] with some modifications. In a typical 30 μl reaction, histone octamer (12.5 pmol) was preincubated for 10 min at 37 °C with 25–50 pmol yeast Nap1 (yNap1) or full-length Scm3 or Scm3 63–189 in a buffer composed of 10 mM Tris-HCl pH 7.5, 200 mM NaCl, 0.6 mM EDTA, 55 μg ml −1 BSA, 10% glycerol, 0.2 mM DTT. A circular-relaxed plasmid or linear DNA (1.2 μg) was added to the reaction and incubated at 37 °C for 2 h. For chromatin assembly on circular-relaxed plasmid, topoisomerase I was added to the reaction and further incubated for 1 h. Assembly was analysed by gel-shift, sucrose gradient sedimentation, DNA supercoiling assay and MNase digestion, as described below. Chromatin purification by sucrose gradient sedimentation Nucleosomes were reconstituted by histone chaperone-mediated chromatin assembly or salt dilution onto a linear 561-bp DNA (with three 147-bp '601' sequence separated by 60 bp of linker DNA), 207-bp CEN3, 5S or 601 DNA. About 100 μl of the reconstituted chromatin samples (concentrated when needed) were loaded onto a 10 ml 5–25% sucrose gradient (in 25 mM Tris-HCl; 7.5, 1 mM EDTA, 1 mM β-Me, 100 mM NaCl) and spun for 18 h at 28,000 r.p.m. at 4 °C in a Beckman SW 41 Ti rotor (Beckman Coulter). The gradients were fractionated by taking out 200 μl from the top and fractions were analysed by 5% native PAGE or 4–12% Bis-Tris SDS–PAGE (Bio-Rad). DNA supercoiling assay Nucleosomes were assembled onto a relaxed circular plasmid (pBR322 or pCR2.1–4 (CEN3+CEN6)) using histone chaperone (yNap1, Scm3 or Scm3 63–189 )-mediated chromatin assembly approach, as described above. The plasmid pCR2.1–4(CEN3+CEN6) contains four copies of CEN3 and CEN6 DNA (a gift from the Henikoff Laboratory). Briefly, histone octamer was preincubated with yNap1, Scm3 or Scm3 63–189 . A relaxed circular plasmid was added and the reaction was incubated for 2 h at 37 °C. A volume of 8 U wheat germ topoisomerase I (Promega) was added and the reaction was incubated at 37 °C for 1 h. The reaction was stopped and deproteinized by adding 0.5% SDS and 0.2 mg ml −1 proteinase K and incubating at 50 °C for 30 min. The DNA extracted was analysed for supercoiling on a 1% agarose gel. Negative and positive plasmid supercoiling was distinguished by running the agarose gel in presence of 1–2 μg ml −1 chloroquine [42] , and by two-dimensional gel analysis in which the samples were run without cholorquine followed by electrophoresis in the second dimension in the presence of 10 μg ml −1 chloroquine [43] . Micrococcal nuclease mapping of nucleosomes Cse4-nucleosomes and canonical nucleosomes were reconstituted onto a 147-bp 601 DNA by salt dilution. Alternatively, reconstitutions were done on a linearized pBR322 plasmid DNA by yNap1-mediated chromatin assembly protocol. The nucleosome samples (reconstituted onto ∼ 5 μg DNA) were digested with MNase (4,000 gel units; NEB) for the indicated times (in Supplementary Fig. S3 ) and quenched by adding EDTA to final concentration of 50 mM. The samples were deproteinized as described above, separated on a 5% native PAGE. Unzipping single DNA molecules in an optical trap Both the forward and reverse nucleosomal DNA templates ( Supplementary Table S1 ) were prepared using published methods [34] , [44] . Cse4- and Sc-nucleosomes were assembled from recombinant yeast histones using salt dialysis. Nucleosomal DNA templates were unzipped using methods similar to those previously described [34] , [44] ( Supplementary Fig. S4 ) under the following buffer condition: 10 mM Tris-HCl (pH 7.5), 1 mM EDTA, 100 mM NaCl, 1 mM DTT, 3% (v/v) glycerol, 0.02% (v/v) Tween-20, 2 mg ml −1 BSA. Size-exclusion chromatography–multiangle light scattering A volume of 100–120 μl of 1–2 mg ml −1 nucleosomes reconstituted on 147-bp 601 DNA were loaded onto a Sephadex 200 (24 ml, GE Healthcare) size-exclusion column at a flow rate of 0.3 ml min −1 using an ÄKTA purifier HPLC system (GE Healthcare). The column was connected to a Dawn Heleos II (Wyatt Technologies) multiangle light scattering instrument, followed by a REx refractive index detector (Wyatt Technologies). To determine the concentration of the nucleosomes a differential index of diffraction (d n /d c ) of 0.175 was used. Small-angle X-ray scattering SAXS data were collected at the advanced light source beamline 12.3.1 and at the Stanford Synchrotron Radiation Light Source (SSRL) BL4-2. Nucleosome solutions identical to those used in SEC–MALS were prepared at 1–8 mg ml −1 in buffer composed of 25 mM Tris-HCl pH 7.5, 1 mM EDTA and 0.2 mM tris (2-carboxyethyl) phosphine. Exposure series of 2, 10 and 2 s were performed at the advanced light source to rule out radiation damage. Data for the reference buffer were collected with the same time series for subsequent intensity-corrected background subtraction and radial averaging of all images. At SSRL, ten 1 s exposures were collected in different spots of a capillary containing the sample. The data were analysed by SasTool and the exposures, which were significantly different, were excluded. Exposures were averaged and buffer scattering was subtracted using SasTool. Data were processed by PRIMUS [45] . Guinier, Porod and Kratky analyses were performed with the same programme. Maximum particle dimensions were determined by indirect Fourier transform with GNOM [46] . Particle reconstructions were performed with the program DAMMIN [47] . Ten reconstructions were averaged and superimposed [48] . Molecular envelopes were constructed with Situs [49] and displayed with VMD [50] . How to cite this article: Dechassa, M. L. et al . Structure and Scm3-mediated assembly of budding yeast centromeric nucleosomes. Nat. Commun. 2:313 doi: 10.1038/ncomms1320 (2011).